Magnetophoretic circuits for digital control of single particles and cells The ability to manipulate small fluid droplets, colloidal particles and single cells with the precision and parallelization of modern-day computer hardware has profound applications for biochemical detection, gene sequencing, chemical synthesis and highly parallel analysis of single cells. Drawing inspiration from general circuit theory and magnetic bubble technology, here we demonstrate a class of integrated circuits for executing sequential and parallel, timed operations on an ensemble of single particles and cells. The integrated circuits are constructed from lithographically defined, overlaid patterns of magnetic film and current lines. The magnetic patterns passively control particles similar to electrical conductors, diodes and capacitors. The current lines actively switch particles between different tracks similar to gated electrical transistors. When combined into arrays and driven by a rotating magnetic field clock, these integrated circuits have general multiplexing properties and enable the precise control of magnetizable objects. One of the main goals of lab-on-a-chip research is to develop generic platforms for manipulating small fluid droplets, colloidal particles and single cells with the flexibility, scalability and automation of modern-day computer circuits. Single-cell arrays represent one high impact application of lab-on-a-chip tools, which are increasingly being adopted to evaluate rare biological responses in small-cell subsets that are overlooked by the ensemble averaging approaches of traditional biology. Improved understanding of these rare cellular responses can profoundly impact the development of vaccines and pharmaceuticals for curing infectious diseases and cancer [1] , [2] ; however there are few existing techniques with the scale and flexibility to unmask single-cell heterogeneity and pave the way for new medical breakthroughs [3] , [4] , [5] , [6] , [7] . In particular, there is an urgent need for tools to organize large arrays of single cells and single-cell pairs, evaluate the temporal responses of individual cell and cell-pair interactions over long durations, and retrieve specific cells from the array for follow-on analyses. The desired capabilities of single-cell arrays bear strong resemblance to random access memory (RAM) computer chips, including the ability to introduce and retrieve single cells from precise locations of the chip (writing data), and query the biological state of specified cells at future time points (reading data). Existing particle handling tools based on hydrodynamic [8] , [9] , [10] , [11] , optic [12] , [13] , [14] , [15] , [16] , [17] , [18] , electric [19] , [20] , [21] , [22] and magnetic [23] , [24] , [25] , [26] , [27] , [28] , [29] , [30] , [31] , [32] , [33] , [34] , [35] , [36] trapping forces can achieve parts of this desired functionality; however, no single technique to our knowledge encompasses the scalability, flexibility and automation that allows single-cell chips to perform with the level of integration of computer circuits. Our approach has significant similarities with magnetic bubble memory technology [37] , which was originally developed to store memory and implement logic through the precise manipulation of ‘magnetization bubbles’ in iron garnet films. Previous works demonstrated that magnetization bubbles could be moved along specific tracks and into desired storage locations by controlling the electrical and magnetic circuitry patterned on top of the garnet films. Magnetic patterns were used to establish a network of highways to move the magnetization bubbles in controlled directions along the pathways of minimum magnetic energy. Current lines were used to switch the bubbles between different highways and store them locally as digital memory. Here, we use a combination of magnetic patterns and current lines to instead control an aqueous suspension of magnetic particles and magnetic-nanoparticle-labelled cells that behave like magnetization bubbles suspended in thin fluid films. The magnetic patterns are used to create passive circuitry analogous to the lumped element conductors, capacitors and diodes of electronic circuits. The current lines are used to establish active circuitry for switching particles and cells between different tracks. When combined together into small arrays, we demonstrate a scalable platform with general multiplexing properties, thereby paving the way for the development of digital circuitry for parallelized control of matter. Magnetic-microparticles and magnetic-nanoparticle-labelled single cells can be reasonably approximated as magnetic point dipoles if they are exposed to weakly inhomogeneous magnetic field distributions on the length scale of the particle. In such cases, the magnetic objects are moved towards the nearest locations of the instantaneous minima of the magnetostatic potential energy that occurs where the local substrate field is parallel to the external field. By shifting the energy minima across the substrate in a programmable manner, the trajectory of single particles can be precisely controlled. If the magnetic field distribution is modulated in time at a sufficiently slow rate, a simple model can demonstrate the similarity between current of magnetic particles and Ohm’s law for electrical circuits, thereby providing motivation for pursuing more complex circuit analogies. The magnetostatic potential energy of a spherical superparamagnetic particle with linear volumetric susceptibility, χ v , in a space- and time-varying magnetic field B is given by: where, V is the volume of the particle, μ 0 is the vacuum permeability and B = B ext + B sub is the total magnetic field generated at the particle centre, which is the sum of a uniform rotating external field, B ext ( t ), and a space–time-varying substrate field, B sub ( r , t ). The local field reaches a maximum at locations where the external field adds to the local substrate field (when the in-plane component of B sub is instantaneously parallel with B ext ), and manifests as a potential energy minimum because of the field squared dependence. Conversely, when the local substrate field partially cancels the external field (when the in-plane component of B sub is instantaneously antiparallel with B ext ), the local potential energy is at a maximum and manifests as a local energy barrier. We intentionally design an asymmetry in the substrate periodicity so that the energy minima can be moved smoothly along desired pathways. We achieve this with a geometry of linearly magnetizable disks, whose magnetization attempts to synchronize with the rotating field direction. The lack of strong hysteresis of the magnetic patterns ( Supplementary Fig. 1 ) justifies this linear approximation. From classical magnetostatics [39] , it is well known that the locations of energy minimum for linear magnetizable systems will occur at positions where the outward normal of the film curvature is aligned parallel to the external field (depicted as the blue regions in simulations of Figs 1 , 2 , 3 , 4 , 5 ). By rotating the external magnetic field in-plane, the locations of the energy minima are continuously shifted around the perimeter of the disk. For substrates consisting of a linear array of half disks connected by linear segments, the motion of the energy minima shifts continuously from one half disk to the next, moving exactly two disk periods, D , for each cycle of the rotating field. The particle transport process is thus similar to a ratchet (or step motor) that transports objects along controlled directions in discrete steps. Here, the local magnetic energy minima can be conceptualized as the nodes in the ratchet. 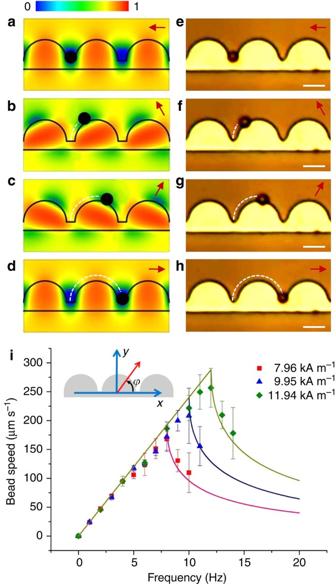Figure 1: Particle conduction. The potential energy landscape for a 2.8-μm-diameter magnetic bead with magnetic susceptibility ofχv=0.65 is shown as it moves around the half-disk track (10-μm diameter, 100-nm-thick NiFe permalloy film) at the external field angles ofϕ=180°, 120°, 60° and 0°. Its motion in a clockwise 7.96 kA m−1rotating field is presented ina–d. Blue and red colours designate the energy minima and maxima, respectively. Corresponding experimental images for the magnetic bead trajectory are shown as the dotted white line ine–h. The red arrows denote the instantaneous magnetic field direction. The velocity versus frequency relationship for the bead motion is presented inifor rotating field strengths of 7.96, 9.95 and 11.94 kA m−1. A schematic of the field angle relative to the track is shown in the inset. The average particle velocity is determined from the time required to travel across 10 periods of the magnetic track, represented as the average (square data point) and s.d. (error bars). The theoretical fit represents an analytical solution to the nonlinear oscillator. The multiplication factor for colour bar is 1.6 × 105kBT. Scale bars, 5 μm. Figure 1: Particle conduction. The potential energy landscape for a 2.8-μm-diameter magnetic bead with magnetic susceptibility of χ v =0.65 is shown as it moves around the half-disk track (10-μm diameter, 100-nm-thick NiFe permalloy film) at the external field angles of ϕ =180°, 120°, 60° and 0°. Its motion in a clockwise 7.96 kA m −1 rotating field is presented in a – d . Blue and red colours designate the energy minima and maxima, respectively. Corresponding experimental images for the magnetic bead trajectory are shown as the dotted white line in e – h . The red arrows denote the instantaneous magnetic field direction. The velocity versus frequency relationship for the bead motion is presented in i for rotating field strengths of 7.96, 9.95 and 11.94 kA m −1 . A schematic of the field angle relative to the track is shown in the inset. The average particle velocity is determined from the time required to travel across 10 periods of the magnetic track, represented as the average (square data point) and s.d. (error bars). The theoretical fit represents an analytical solution to the nonlinear oscillator. The multiplication factor for colour bar is 1.6 × 10 5 k B T. Scale bars, 5 μm. 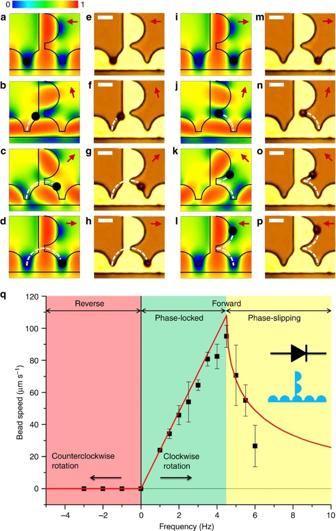Figure 2: Particle rectification. The potential energy landscape in a clockwise 7.96 kA m−1rotating field in the forward-biased diode mode is shown when the external field has angular orientation ofϕ=180°, 105°, 45° and 0° as presented ina–d. The red arrows denote the instantaneous external field direction. The blue energy minima correspond to the particle locations in the experimental images ofe–h. The potential energy landscape for the reverse conditions for field angles ofϕ=0°, 75°, 135° and 180° is presented ini–lalong with the associated experimental images inm–p. The velocity versus frequency relationship for the matter rectifier is presented inq. The average particle velocity is determined from the time required to travel across 10 periods of the magnetic track, represented as the average (square data point) and s.d. (error bars). The theoretical fit represents an analytical solution to the nonlinear oscillator. The multiplication factor for colour bar is 1.6 × 105kBT. Scale bars, 5 μm. Full size image Figure 2: Particle rectification. The potential energy landscape in a clockwise 7.96 kA m −1 rotating field in the forward-biased diode mode is shown when the external field has angular orientation of ϕ =180°, 105°, 45° and 0° as presented in a – d . The red arrows denote the instantaneous external field direction. The blue energy minima correspond to the particle locations in the experimental images of e – h . The potential energy landscape for the reverse conditions for field angles of ϕ =0°, 75°, 135° and 180° is presented in i – l along with the associated experimental images in m – p . The velocity versus frequency relationship for the matter rectifier is presented in q . The average particle velocity is determined from the time required to travel across 10 periods of the magnetic track, represented as the average (square data point) and s.d. (error bars). The theoretical fit represents an analytical solution to the nonlinear oscillator. The multiplication factor for colour bar is 1.6 × 10 5 k B T. Scale bars, 5 μm. 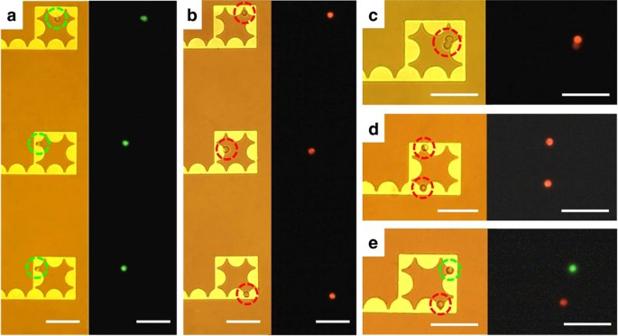Figure 3: Local storage of magnetically labelled single cells. Bright-field and fluorescent images of (a) single T lymphocytes and (b) B lymphocytes trapped in individual apartments are shown. Real-time analysis of biological process, such as mitosis, can be observed inc. A homogeneous pairing of (d) B lymphocytes and a heterogeneous pairing (e) of a B- and T lymphocytes can be trapped in a single apartment, demonstrating the ability to arrange single-cell pairs. Scale bars, 40 μm. Full size image Figure 3: Local storage of magnetically labelled single cells. Bright-field and fluorescent images of ( a ) single T lymphocytes and ( b ) B lymphocytes trapped in individual apartments are shown. Real-time analysis of biological process, such as mitosis, can be observed in c . A homogeneous pairing of ( d ) B lymphocytes and a heterogeneous pairing ( e ) of a B- and T lymphocytes can be trapped in a single apartment, demonstrating the ability to arrange single-cell pairs. Scale bars, 40 μm. 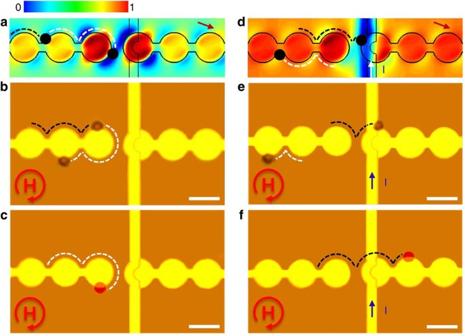Figure 4: Type I transistor for local switching of single particles and cells. A small gap fabricated between two adjacent magnets allows a single particle to be selectively transported in the positive or negativexdirection based on whether a 100-mA current applied is turned ON or OFF. Partsa–cshow the potential energy landscape, and the experimental trajectory (white dotted line) of a single particle or cell when the current line is OFF. Partsd–fshow the same conditions when the current is ON. The merger of the energy minima causes the particles to move across the gap only when the current line is ON. The red arrows denote the instantaneous external field direction. The multiplication factor for colour bar is 1.6 × 105kBT. Scale bars, 20 μm. Full size image Figure 4: Type I transistor for local switching of single particles and cells. A small gap fabricated between two adjacent magnets allows a single particle to be selectively transported in the positive or negative x direction based on whether a 100-mA current applied is turned ON or OFF. Parts a – c show the potential energy landscape, and the experimental trajectory (white dotted line) of a single particle or cell when the current line is OFF. Parts d – f show the same conditions when the current is ON. The merger of the energy minima causes the particles to move across the gap only when the current line is ON. The red arrows denote the instantaneous external field direction. The multiplication factor for colour bar is 1.6 × 10 5 k B T. Scale bars, 20 μm. 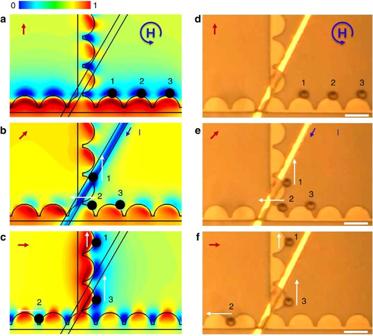Figure 5: Type II transistor for particle rectification reversal. A diagonal current line superimposed on the T-junction is used to selectively transfer single particles across the junction. Partsa,dshow the potential energy landscape and its associated experimental image when the current is OFF for three particles approaching the junction. Partsb,eshow the potential energy landscape and its associated experimental image when the current is ON, after the first particle has passed, but before the second and third particles have reached the junction. Partsc,fshow the potential energy landscape and its associated experimental image when the current is OFF. Only the second particle crossed the junction in the negativexdirection, whereas the first and third particles are moved in the positiveydirection. The red arrows depict the external field direction. The white arrows depict the future direction of the magnetic beads. The multiplication factor for colour bar is 1.6 × 105kBT. Scale bars, 20 μm. Full size image Figure 5: Type II transistor for particle rectification reversal. A diagonal current line superimposed on the T-junction is used to selectively transfer single particles across the junction. Parts a , d show the potential energy landscape and its associated experimental image when the current is OFF for three particles approaching the junction. Parts b , e show the potential energy landscape and its associated experimental image when the current is ON, after the first particle has passed, but before the second and third particles have reached the junction. Parts c , f show the potential energy landscape and its associated experimental image when the current is OFF. Only the second particle crossed the junction in the negative x direction, whereas the first and third particles are moved in the positive y direction. The red arrows depict the external field direction. The white arrows depict the future direction of the magnetic beads. The multiplication factor for colour bar is 1.6 × 10 5 k B T. Scale bars, 20 μm. Full size image The particle currents can be approximated mathematically by modelling the tangential force, F t , of a magnetic particle around the circumference of a thin disk-shaped micro-magnet: where f(η,θ) is the forcing magnitude, which depends on the external field as well as geometric and material properties. The coordinates η and θ represent the position of the particle centre in oblate spheroid coordinates, which is the most natural coordinate system to model the particle trajectory around a thin disk, and leads to convenient analytical expressions. In equation (2), the parameter ψ represents the angular location of the particle relative to the horizontal axis, and ω ext is the frequency of the rotating external field. When re-written in the travelling reference frame by using the change of variable, Ω = ψ − ω ext t , the dynamics is equivalent to the ratchet motion of a non-uniform oscillator: d Ω /d t =– ω ext +ω c sin(2 Ω ), where ω c = f ( η,θ )/6 πη f R p D is the maximum driving frequency that satisfies the linear regime of Ohm’s law for a particle of radius, R p , in a fluid of viscosity, η f . The parameter, Ω , represents the phase lag of the bead behind the nearest energy minima. For subcritical frequencies ( ω ext ≤ω c ), the phase lag is small but constant (2 Ω≤π/ 2), allowing the particle find a stable phase where d Ω /d t =0, called the phase-locked regime. In this regime, the particle moves deterministically with time-averaged velocity: where is the sense of the rotating external field, and is the unit vector pointing away from the centre of a given disk. The linear relationship between frequency and magnetic particle current ( I b =ω ext /R b ) behaves analogously to Ohm’s law ( I e =V/R e ), in which the resistance, R b , is inversely related to the pattern periodicity, 2 D . At higher frequencies ( ω ext >ω c ), the particle’s phase lag is no longer able to satisfy the inequality 2 Ω ≤ π /2 because of the increase in viscous force beyond a critical threshold, which cause the particle to periodically slip out of a given potential energy minima into the nearest adjacent minima. The resulting phase-slipping motion is characterized by oscillating attractive and repulsive forces on the particle and an overall decrease in the particle’s time-averaged velocity, as well as periodic changes in direction. Conductors for reversible current flow Figure 1 presents the particle trajectory as a function of the time-varying field angle, φ=ω ext t , where increasing angles correspond to a counter-clockwise rotating field. Simulations of the potential energy distribution ( Fig. 1a–d ) compared with the experimental trajectory ( Fig. 1e–h ) demonstrate that the particle position is correlated to the shifting regions of potential energy minima (blue). The particles move along the upper section of the track because it has the deepest energy minima. The linear segment connecting adjacent magnets provides an energy barrier that confines the local energy minima to one side of the magnetic track. For sufficiently low driving frequencies, the particles move exactly two array periods for each complete cycle of field rotation, demonstrating the linear relationship between frequency and magnetic particle current for the phase-locked regime ( Fig. 1i ). Clockwise field rotation leads to particle motion along the positive x direction, whereas counter-clockwise rotation produces motion along the negative x direction ( Supplementary Movie 1 ). The asymmetry in the track design is essential for achieving a net particle current. If the track were designed with full disks instead of half disks, then the particles confined to the lower portion of the track would move in the opposite direction of the particles on the upper portion, thereby negating net current flow. At higher frequencies, the particles enter the phase-slipping regime, and the analogies with Ohm’s law breaks down ( Fig. 1i ). Rectifiers for irreversible current flow Rectification is accomplished by introducing additional asymmetry in the conductor paths, such as by joining two magnetic tracks in a T-shaped junction ( Fig. 2 ). In the forward-biased mode ( Fig. 2a–h ), the particle initially moves from left to right on the horizontal track in the positive x direction. When the particle reaches the T-junction, the two potential energy minima on either side of the junction merge together (see the transition of the two blue regions in Fig. 2a into one blue region in Fig. 2b ), which permits the particle to jump over the linear vertical segment. After surmounting this barrier, the particle continues its horizontal path along the positive x direction in sync with the rotating field. Alternatively, if a particle were initially moving in the negative y direction on the vertical track, then it also turns toward the positive x direction at the T-junction. This asymmetric track design ensures that regardless of the origin of the particle currents, matter will eventually flow along the positive x direction in a clockwise rotating field. An example of the reversed bias rectification mode can be observed in the counter-clockwise driving field ( Fig. 2i–p ), in which the particle moves along the negative x direction of the horizontal track. When the particle reaches the T-junction, the single energy minima ( Fig. 2j ) splits into two blue/green metastable energy minima ( Fig. 2k ). See Supplementary Figs 2 and 3 for more detailed illustration of the energy pathways. The slightly red region directly on top of the vertical segment of the magnetic track in Fig. 2k depicts a local energy barrier that prevents the particle from crossing over the linear vertical segment. Instead, the particle follows the deeper energy minimum that moves in the positive y direction and enforces the asymmetry of the conduction mechanism. The overall effect is that particles can conduct along the positive x direction in a clockwise rotating field, but cannot conduct along the negative x direction in a counter-clockwise rotating field. The irreciprocal motion of the particle pathway is also depicted in Supplementary Movie 2 . The velocity versus frequency relationship for the matter rectifier is presented in Fig. 2q . Note that the critical frequency that defines the transition between the phase-locked and phase-slipping regimes is lowered for the diode relative to the conductor track of Fig. 1 , owing to the modified energy landscape of the T-junction. Capacitors for local storage of single particles and cells Rectification and conduction pathways can be geometrically arranged in closed loops to store small single particles and cells in well-defined spatial regions, operating in a manner similar to an electrical capacitor. Figure 3a shows an array of magnetic conduction tracks and square apartments that are configured such that the T-junction entry way is in the forward bias mode and allows particles or cells to enter the apartment. In a clockwise driving field, single immune cells labelled with 50-nm magnetic nanoparticles are moved into the apartments, where they subsequently remain trapped in a closed spatial orbit. Upon reversing the field rotation, the cells remain trapped in their apartments because of the reverse bias of the diode junction ( Supplementary Movie 3 ). By this mechanism, single T- and B-cell lymphocytes ( Supplementary Movie 4 ) can be arrayed in individual apartments that allows for long-term analysis of single cells and visualization of biological processes such as cell mitosis ( Fig. 3d ). The ability to trap pairs of cells in individual apartments, including a homogeneous pair of B-lymphocyte cells ( Fig. 3e ) or a heterogeneous pair of B- and T-lymphocyte cells ( Fig. 3f ), can serve as a platform for studying single cell–cell communication. Type I transistors for local matter switching The ability to perform selective operations on a specific particle or cell within a large array can be accomplished by combining passive transport elements with locally addressible active elements to switch particles along different tracks as well as into (or out of) a local apartment. Here we show one mechanism for switching a particle between two different pathways by creating a controlled gap between two disks in the magnetic track. A current line placed at one edge of the gap generates a competing magnetic field that tunes the local energy landscape and switches the particle between conductive and non-conductive states. This transport behaviour has analogies with the action of a gate electrode in switching currents at a semiconducting junction. When the current is OFF, the energy landscape is a bistable double-well potential, which can be visualized as the two blue energy minima regions on either side of the gap in Fig. 4a . The double-well potential restricts the particle to one side of the gap and reverses its direction of motion (white dotted in line in Fig. 4b,c ). When the 100 mA current is ON, the two bistable energy minima merges into a single energy minimum that causes the gap to become conductive and moves the particles across the gap along the positive x direction (black dotted line in Fig. 4e,f ). By timing the current pulses in sync with the rotating magnetic field clock, it is possible to selectively transfer one particle while preventing another particle from crossing the gap ( Fig. 4b,e and Supplementary Movie 5 ). Selective operations can also be performed on single cells ( Fig. 4e,f and Supplementary Movie 6 ). In Fig. 4e,f , pseudo-coloring is used to increase the contrast of the cell relative to the background. Type II transistors for local matter switching In some applications, it is necessary to retrieve a particle or cell from confinement to perform genome sequencing or follow-on analysis. This functionality requires the ability to reverse the rectifier bias and allow a single particle or cell to escape from the apartment. Here we place a diagonal current line oriented at a 60° angle relative to the horizontal axis on the opposite side of the rectifier junction that allows the particle to escape the apartment when a gate current is applied. When the 100 mA current is ON, the bistable energy minima on either side of the junction of Fig. 5a merge together into a single energy minimum on top of the junction, as shown in Fig. 5b . The subsequent motion of the energy minima of Fig. 5c is modulated by the applied current that removes the energy barrier of Fig. 3k and increases the depth of the energy minima on the opposite side of the rectifier junction. After passing the junction, the particle continues along the negative x direction of the horizontal track. Owing to the deterministic nature of particle transport, the switching process can be synchronized with the external field clock to permit the second particle, but not the first or third particle, to move across the junction. The paths of the three particles are illustrated with the white arrows and are shown more clearly in Supplementary Movie 7 for single particles and Supplementary Movie 8 for single cells. Multiplexed operations The 3 × 3 array of Fig. 6 demonstrates one potential multiplexing strategy, in which three horizontal and three vertical current lines are used to control the arbitrary deposition of up to nine particles. In this implementation, when the top row current line is ON while keeping the bottom two row current lines OFF ( Fig. 6a ), particles will be transported along the top row magnetic track. If the right column current line is also applied, then the particle is eventually deposited in the upper-right apartment of Fig. 6a . By timing the current impulses in columns 1 and 3, this general procedure is used to deposit particles 1 and 2 in the left and right apartments of the top row. Next, particles 3 and 4 are deposited in the left and right apartments of the bottom row ( Fig. 6c ). Finally, particle 5 is deposited in the middle apartment of the middle row, thereby generating a particle pattern in the shape of an ‘X’. Supplementary Movie 9 depicts the particle deposition process, and Supplementary Fig. 4 shows examples of other particle patterns that can be deposited with this approach. Owing to the deterministic nature of this transport mechanism, these circuits can perform timed operations on single particles and cells with knowledge of only their initial conditions (position at some previous time) and the number of magnetic field clock cycles that have passed since the previous operation. 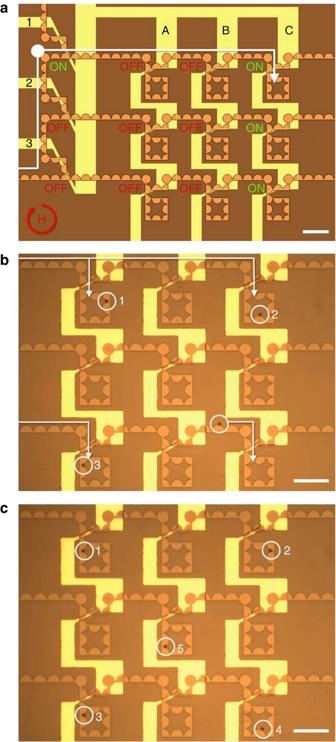Figure 6: Multiplexed circuits for arraying single particles. An integrated circuit containing a 3 × 3 array of apartments is overlaid with three horizontal row switches and three vertical column switches in multiplexed format. Partashows the basic methodology for moving a single particle to the upper-right apartment by applying current only to the top row (1) and right column (C) current lines. All other current lines are in the OFF state and are not populated with single particles. Partbshows the positions of the first three deposited particles and the destination of a fourth particle. Partcshows the array populated with an ‘X’ pattern of single particles. Scale bars, 60 μm. Figure 6: Multiplexed circuits for arraying single particles. An integrated circuit containing a 3 × 3 array of apartments is overlaid with three horizontal row switches and three vertical column switches in multiplexed format. Part a shows the basic methodology for moving a single particle to the upper-right apartment by applying current only to the top row (1) and right column (C) current lines. All other current lines are in the OFF state and are not populated with single particles. Part b shows the positions of the first three deposited particles and the destination of a fourth particle. Part c shows the array populated with an ‘X’ pattern of single particles. Scale bars, 60 μm. Full size image Bioselective logic In addition to the basic circuit elements and integrated circuits presented in Figs 1 , 2 , 3 , 4 , 5 , 6 , it is also possible to exploit other dynamic regimes to achieve bioselective functionality. The example depicted in Fig. 7 indicates a methodology for tuning the gap junction to be non-conductive for single magnetic particles but conductive for single magnetic particles attached to single T-lymphocyte cells. This sorting mechanism exploits the high-frequency regime of the nonlinear oscillator phenomena described in equation (2), which allows for particles to transition between the phase-locked and phase-slipping states of the ratchet. The switching mechanism exploits the lag of a particle that trails behind the phase of the translating energy minima by an amount Ω = ψ − ϕ . The specific phase lag depends on the radius of curvature of the track, viscous friction coefficient of the particle and the magnetic properties of the system. 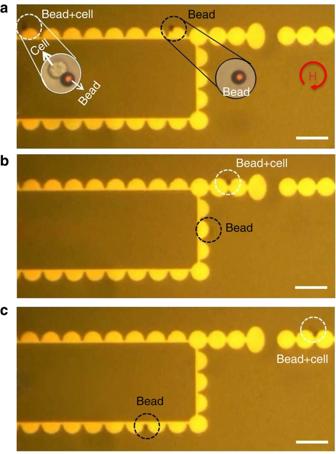Figure 7: Bioselective logic for separating particles. A small gap fabricated between two magnetic patterns is used to selectively separate a single bead (black) from a bead+cell complex (white). The gap is designed with an elliptical pattern at the left edge, which tunes the dynamic range of particle motion. Partashows the state before the bead and bead+cell have reached the junction. Partbshows a time immediately before the bead+cell, but after the single bead, has passed the junction. Partcshows the state after both the bead and bead+cell have passed the junction. The bead+cell complex is transferred across the gap, whereas the single bead is not. The operating frequency is 2 Hz. Scale bars, 40 μm. Figure 7: Bioselective logic for separating particles. A small gap fabricated between two magnetic patterns is used to selectively separate a single bead (black) from a bead+cell complex (white). The gap is designed with an elliptical pattern at the left edge, which tunes the dynamic range of particle motion. Part a shows the state before the bead and bead+cell have reached the junction. Part b shows a time immediately before the bead+cell, but after the single bead, has passed the junction. Part c shows the state after both the bead and bead+cell have passed the junction. The bead+cell complex is transferred across the gap, whereas the single bead is not. The operating frequency is 2 Hz. Scale bars, 40 μm. Full size image In the example given in Fig. 7 , the elliptical element at the junction is used to uniformly lower the critical frequency of the system and adjust the dynamic ranges of the two particles. Owing to the larger viscous friction coefficient for the bead+cell complex, its critical frequency, ω c1 , is lower than the critical frequency of the single bare bead, ω c2 , (that is, ω c1 <ω c2 ). Thus, there exists an operating frequency, ω ext that is higher than the critical frequency of the bead+cell complex, but lower than the critical frequency of the single bare bead, (that is, ω c1 <ω ext <ω c2 ). By satisfying these conditions, the bead+cell complex is in the phase-slipping regime and is ejected out of the local energy minima into an adjacent energy minimum on the opposite side of the gap via a repulsive force [38] . However, the bare bead is in the phased-locked regime and remains trapped inside its local energy minimum on the same side of the gap ( Supplementary Movie 10 ). This mechanism can separate multiple different particles based on the size of their biological payload, as well as by tuning the size of the ellipse and the magnetic system properties. The phase-slipping regime of ratchets has previously been used to separate different particles based on size [24] ; however, to our knowledge it has not been used to control the overall direction of different particles along two separate tracks, allowing for more flexible implementation as a bioselective logic mechanism. Here we have demonstrated scalable integrated circuits for transporting magnetic particles and single cells along programmable pathways in microfluidic environments. Towards this goal, we have arranged a combination of conductors, rectifiers, capacitors and transistors in multiplexed format to demonstrate the basic skeleton for executing massively parallel operations with a mininum number of control wires. The N × N crossbar array used in our multiplexing architecture is inspired by the ‘word’ line and ‘bit’ line architecture of static RAM circuits. If the circuitry is further optimized, we estimate these arrays can store more than 10 6 cells in −2 based on the 10-μm lower limit of a typical cell diameter. Our clock cycles are probably limited to the 1–10 Hz range because of the relatively high fluid viscosity and low magnetic forces. Although this performance pales in comparison with the speed of modern computer circuits, it is possible to increase the scale of operations by partitioning this circuit into multicore processor format. Based on these considerations, it is not unreasonable to suggest the possibility of performing more than 10 6 single-cell operations in an hour, which is on the relevant timescale of many cellular processes. This system is thus highly relevant to the burgeoning field of single-cell informatics that requires programmable systems to automate the separation of different cells either actively or passively; place single cells and single-cell pairs into large arrays; characterize their cellular interactions over long times; and selectively retrieve single cells at future time points for follow-on analyses. Materials Superparamagnetic particles of 2.8-μm diameter (Dynabeads M-280) and superparamagnetic beads of 4.5-μm diameter (Dynabeads mouse Pan T; Thy1.2) were purchased from Invitrogen, Grand Island, NY, USA. Magnetic nanoparticles of 50-nm diameter conjugated with CD90.2 (Thy1.2; T lymphocytes) and CD45R (B220; B lymphocytes) were procured from Miltenyi Biotec Inc., Auburn, CA, USA. Silicon wafers coated with 200 nm of SiO 2 were obtained from Wafermart. Photoresist (AZ 5214-E) and developer was purchased from AZ electronic materials. Polydimethylsiloxane (Sylgard 184) was procured from Dowhitech Silicone. All chemicals used for cell media were obtained from Sigma-Aldrich. Pan T-cell and Pan B-cell isolation kit were procured from Miltenyi Biotec Inc. Calcein AM green and red/orange was purchased from Invitrogen. Magnetic circuit design Soft permalloy (Ni 82.6 Fe 17.4 ) patterns of 100 nm thickness are combined with 200-nm thick conductive Au patterns fabricated on silicon or glass substrates using conventional photolithographic lift-off method separated by a 150-nm insulating layer of SiO 2 . The magnetic patterns consisted of an array of half disks with either 5 or 10-μm radius, connected by magnetic segments 2 μm in length. Magnetic film properties were measured by vibrating sample magnetometry (Lakeshore 7400). External rotating magnetic field was produced by passing current through pairs of solenoid coils with ferrite cores controlled by LabVIEW (National Instruments). The sense of field rotation was adjusted by applying a phase difference, δ = ±90° between the orthogonal coils with field magnitudes ranging from 0 to 15.9 kA m −1 . A constant current source was controlled by LabVIEW to provide 100 mA DC pulses through the wires to achieve particle switching and exiting from the apartment. Data analysis Particle motion was tracked by video microscopy using a IMC-1040FT video camera. The average particle velocities were determined from the time required to travel across 10 pattern periods. The average and s.d. of the velocity data are plotted in the figures. Nanoparticle–lymphocytes conjugation Lymphocytes were isolated from the spleens of C57BL6 mice (KOATECH, Pyeongtaek, Korea) by negative magnetic-activated cell sorting using Pan T-cell and Pan B-cell isolation kit, respectively, together with lymphocyte separation columns and Midi-magnetic-activated cell sorting magnets according to the manufacturer’s instructions ( Supplementary Fig. 5 ). The magnetic nanoparticles were immobilized on isolated lymphocytes via interaction between antigen expressed in lymphocytes and corresponding antibody conjugated to magnetic nanoparticles ( Supplementary Fig. 6 ). The T cells and B cells were labelled with calcein dye (green and red/orange, respectively). Bioselective logic experiment The magnetic beads with diameter 4.5 μm were immobilized on isolated T lymphocytes from the spleens of C57BL6 mice via interaction between antigen expressed in lymphocytes and corresponding antibody conjugated to magnetic beads ( Supplementary Fig. 7 ) Finite element method Finite element simulations were performed in Maxwell 3D software (version 12.2, Ansoft), which used experimentally derived material constitutive relationships to model the magnetic field distribution and magnetostatic potential energy. Specifically, we used the experimentally measured magnetization hysteresis curve of thin permalloy film with 100-nm thickness ( Supplementary Fig. 1b ), from which we obtained the saturation magnetization and coercivity value of 668 emu cc −1 and 190 A m −1 , respectively. The potential energy on the magnetic beads was determined according to equation (1), and is plotted as a function of the external field orientation. Analytical model In addition, we developed semi-analytical approximations to represent the magnetic field of thin film patterns in the shape of disks, half disks, and thin strips connected together in serial arrangements. Although the semi-analytical approach comes at the cost of numerical precision, it reduces the computational burden to allow for more computationally feasible trajectory calculations and presentation of potential energy animations. Our first concern was to develop a model for the local magnetic field that is consistent with the shape-induced anisotropy of various film geometries, but without introducing local numerical artefacts. The geometry of thin disks connected together by short strips can be approximately modelled as an overlapping set of paramagnetic ellipsoids and oblate spheroids. This approximation has the advantage of accurately capturing the influence of shape-induced demagnetizing factors on the local magnetization; however, near the overlapping regions this approach introduces spurious magnetic pole distributions that influence the local magnetic fields and forces. At the other end of the modelling spectrum, magnetic thin film patterns exposed to in-plane magnetic fields are commonly approximated as line charges around the perimeter of the patterned film; however, these approximations do not account for shaped-induced demagnetizing factors. Ultimately, we settled on a hybrid model that achieves a semi-self-consistent solution for local magnetization without introducing spurious pole distributions. Although these models represent an approximation to the numerically exact, finite element analyses, they markedly increase the computation speed. The magnetic field of a uniformly magnetized ellipsoid with semi-principal axes of length a , b and c along the x- , y- and z directions, respectively, has previously been derived by Stratton [39] . The analytical expression for the magnetic potential inside and outside a paramagnetic ellipsoid is given by: where ϕ ext and ϕ s represent the uniform external field and ellipsoid potential in the x direction, respectively. The functions , and are one-dimensional orthogonal expansions in the ellipsoidal coordinate system, in which the coordinate ξ can be considered as the radial term, whereas the η and ζ coordinates represent the angular distribution, with a characteristic length scale of R s for the system. The coefficients, C 1 , C 2 and C 3 are determined by matching the boundary conditions of equation (4, 5, 6) which must satisfy the continuity of the magnetic potential and its normal first derivative at the boundary: where ξ=0 represents ellipsoid’s surface and where μ 0 and μ 1 are the magnetic permeability outside and inside the ellipsoid, respectively. Similar equations can be achieved for the external field in the y - and z directions by replacing a in equation (1) with b and c , respectively. Owing to the high magnetic permeability of permalloy material used in experiments, we make the assumption that μ 1 >>μ 0 with the surrounding medium assumed to be vacuum. The metric coefficient is given by: After deriving the matching coefficients C 1 , C 2 and C 3 and inserting them in equations (4, 5, 6, 7, 8), the potentials inside and outside the ellipsoid are determined to be: while p and q take values of 0, ξ and ∞ . Assuming a=b>c , equations (10 and 11) can be solved analytically for the magnetic potential of an oblate spheroid [40] , [41] ; however, ellipsoidal solutions require either tabulated integrals or direct evaluation of the A i components through numerical integration. In experiments, the magnetic tracks are formed from a thin continuous film composed of magnetic disks (or half disks) connected by short linear segments. The ellipsoidal models described above are a good approximation for the field distributions far from the intersections of the disk and linear segments; however, these approximations produce spurious poles at the intersection points that do not match the expected pole distribution of these geometries. In order to reduce these inconsistencies, we further refine our model to approximate the substrate as a continuous line charge spanning the areal perimeter of the magnetic tracks. By matching the line charge model with the ellipsoidal model, we ensure that the shape-induced demagnetizing factors reflect the local magnetization of different parts of the pattern without introducing spurious poles. The advantage of this approach is that the simulation time for calculating the magnetic field of the substrate can be reduced from days to minutes. The magnitude of the line charge density is determined by the local magnetization mismatch across the materials boundary at the edges of the magnetic film. The divergence condition inside uniformly magnetized ellipsoids is represented as a surface charge distribution: where H out and H i n are the fields outside and inside the ellipsoid, respectively, with n representing the local outward normal of the ellipsoid curvature. Since the magnetic patterns of experiment are very high aspect ratio (approximately flat), the majority of magnetic poles are confined to the edges of the ellipsoid, which allow it to be approximated as a line charge with density: where 2 c is the thickness of the film. We use a numerical matching coefficient, γ , in order to match the far field approximation of the line charge model with the ellipsoid model. This matching coefficient is determined by least squares analysis between the volume averaged field of the line charge from equation (14) and the analytical solution for the ellipsoid’s field from equations (10 and 11). In the experimental geometries, the value of γ is found to be 0.124 and 0.0406 for the disk and linear segments, respectively. The linear segments are approximated as a spatially constant line charge, which varies with the time-varying vector product between the field direction and the substrate normal. The disk segments are approximated as a continuously varying line charge density with the maximum occurring at the location where the substrate normal is parallel to the external field. The line charge density of equation (14) varies in time due with angular rotation of the external field, ω ext . By accounting for this time-varying substrate pole density, we obtain an approximation of the magnetic potential by performing one-dimensional integrations over the exterior of the of the magnetic pattern as follows: where represents the distance between an element of the line charge and the observation point. The line charge density, λ ( t ), varies with time and the outward normal of the local pattern curvature, n s . The magnetic field is determined by taking the negative gradient of the magnetic potential. For the active switches, we assume the current lines are infinitely thin compared with the planar dimensions. The magnetic field produced by these sheet currents can be calculated from the Biot–Savart law: where is the magnitude of the local sheet current, and is the location of the observation point, r , relative to the source point, r s . For simplicity, we assume that the sheet currents do not interact with the magnetization patterns, and that the currents are uniformly distributed within the current lines. The magnetic force on particles exposed to this combination of time-varying magnetic fields is approximated as the force of a point dipole in an external field gradient: The force in the vertical direction , F z , is ignored as it is usually <0 and is therefore attractive towards the surface. The moments of the magnetic beads (or magnetized biological particles) are assumed to obey a linear relationship with the fields given by: m = χ v V B/ μ 0 , which is valid for fields kept below the saturation magnetization of 120 Oes for commonly available magnetic beads. For small particles in aqueous fluids, the particle motion is typically modelled with overdamped first order equations of motion. The particle velocity is assumed to be proportional to the magnetic force and inversely proportional to the Stoke’s friction coefficient for a sphere in a quiescent fluid, 6 πη f R p . The particle trajectory is determined by integrating the velocity in a simple forward difference scheme, r i = r i− 1 + v i− 1 Δ t, in which the particle position at the i th timestep, r i , is determined from its position and velocity at the previous timestep, r i− 1 and v i− 1. The timestep, Δ t , is chosen to simultaneously optimize numerical convergence and computational expense. How to cite this article: Lim, B. et al. Magnetophoretic circuits for digital control of single particles and cells. Nat. Commun. 5:3846 doi: 10.1038/ncomms4846 (2014).